Water-mediated deracemization of a bisporphyrin helicate assisted by diastereoselective encapsulation of chiral guests Deracemization is a powerful method by which a racemic mixture can be transformed into an excess of one enantiomer with the aid of chiral auxiliaries, but has been applied only to small chiral molecular systems. Here we report a deracemization of a racemic double-stranded spiroborate helicate containing a bisporphyrin unit upon encapsulation of chiral aromatic guests between the bisporphyrin. The chiral guest-included helicate is kinetically stable, existing as a mixture of right- and left-handed double helices, which eventually undergo an inversion of the helicity triggered by water resulting from the water-mediated reversible diastereoselective B-O bond cleavage/reformation of the spiroborate groups, thus producing an optically-active helicate with a high enantioselectivity. Quantum chemical calculations suggest that the stereospecific CH-π interactions between the porphyrin hydrogen atoms of the helicate and an aromatic pendant group of the chiral guest play a key role in the enhancement of the helical handedness of the helicate. The double-helix is one of the topologically unique structures, which is instantly reminiscent of the DNA double-helix. Hence, the design and synthesis of artificial double helices has become an attractive challenge with implications for sophisticated biological structures and functions [1] , [2] , [3] , [4] , [5] , [6] . Among the double helices prepared so far, helicates, a class of metal-directed self-assembled helical complexes, are the most popular structural motifs since the seminal work by Lehn and co-workers [7] , [8] , [9] , [10] , [11] . The control of its handedness is of key importance for developing one-handed helicates with a specific functionality that involves separation [12] and sensing enantiomers [12] , [13] , [14] and asymmetric catalysis [15] as well as antimicrobial materials [16] . However, double-stranded helicates composed of achiral molecular strands assembled with labile metal ions, such as Cu(I) ions, mostly exist in an equal mixture of interconvertible right- ( P ) and left-handed ( M ) helices and their resolution into the enantiomers remains difficult except for one example [17] . A preferred-handed helicity can be biased in such kinetically labile double-stranded helicates using a chiral template [18] or chiral auxiliaries [19] , [20] , [21] , but the helicates likely lose their optical activities after removal of the chiral template or chiral auxiliaries due to irreversible racemization in solution. This asymmetric transformation of a racemic mixture into a nonracemic one by the presence of chiral species, a typical class of deracemizations [22] , [23] , is known as the Pfeiffer effect [24] , and was first observed in kinetically labile racemic coordination complexes an almost century ago [25] , [26] . Thereafter, this (asymmetric transformation strategy) concept has been applied to a variety of configurationally labile enantiomers [22] , [27] , [28] , [29] including helicates [19] , [20] , [21] and dynamically racemic helical polymers [30] . In contrast to kinetically labile helicates, double- and triple-stranded helicates with a hexa-coordinated, octahedral geometry composed of a substitution-inert metal are kinetically stable and can be readily separated into the enantiomeric helices by traditional resolution in the maximum yield of 50% [10] , [17] , [31] , [32] . Therefore, it is significantly required to develop a versatile method, which enables to quantitatively deracemize a racemic mixture of kinetically labile helicates into kinetically stable helicates with an excess of one enantiomer upon noncovalent interactions with chiral guests. This deracemization technique is an ideal and promising approach to produce an excess of one enantiomer or a nonracemic product in 100% theoretical yield from a racemic mixture [23] , [33] , [34] , [35] , but has been limited to small chiral molecular systems [33] , [34] , [35] except for one example observed in supramolecular helical polymers [36] , which are stereochemically stable but can deracemize via a bond cleavage/reformation process that proceeds in a diastereoselective or enantioselective fashion assisted by chiral catalysts in dynamic kinetic resolutions [37] and chiral hosts or upon crystallization with chiral external forces [35] , [38] , thus producing nonracemic products or enantiomers. In an earlier study, we reported a series of racemic double-stranded helicates consisting of two spiroborate groups bridged by two achiral tetraphenol strands bearing a variety of linkers in the middle [39] . The racemic helicates can be resolved into optically-pure enantiomers by conventional diastereomeric salt formation followed by ion exchange with an achiral ammonium salt [39] , [40] , [41] . The optically-active spiroborate helicates are stable and tolerant toward racemization in aprotic polar solvents, but racemize in the presence of a catalytic amount of acid as a proton source, indicating that the spiroborate helicates possess both dynamic (labile) and static (inert) features toward racemization (Fig. 1b ). Fig. 1 Deracemization and diastereoselective inclusion complexation of double-stranded spiroborate helicates. a Chemical structures of double-stranded bisporphyrin helicates 1 X2 (X = Na + or TBA + ) and their inclusion complexation with achiral ( G1 ) or chiral ( G2 – G8 ) electron-deficient aromatic guests. b , c Schematic representations of water-catalyzed racemization of rac - 1 Na2 ( b ), deracemization of rac - 1 Na2 upon the inclusion complex formation with an enantiopure guest ( c ), and diastereoselective inclusion complexation of racemic guest with left-handed ( M )- 1 TBA2 ( d ) Full size image Here, we show a water-mediated deracemization of a racemic spiroborate helicate containing a bisporphyrin [41] , [42] , [43] , [44] , [45] , [46] unit ( 1 ) [47] (Fig. 1a ) upon diastereoselective encapsulation of an electron-deficient chiral aromatic guest between the porphyrin rings of the racemic helicate (Fig. 1c ) assisted by stereospecific CH–π interactions. The interconversion between the ( P )- and ( M )-helicates takes place through a water-mediated dynamic B–O bond [48] , [49] cleavage/reformation reaction that occurred at the spiroborate moieties in a highly helix-sense selective way, thus producing an optically-active static helicate from a racemic mixture after the removal of water. Synthesis of the helicate and guests The racemic and enantiopure ( P )- or ( M )-bisporphyrin helicates ( rac - 1 Na2 and ( P )- or ( M )- 1 TBA2 , respectively; TBA = tetra- n -butylammonium, Fig. 1a ) were prepared according to a previously reported method [47] . The helicate 1 forms a stable inclusion complex with an electron-deficient planar guest, such as G1 ( 1 Na2 ⊃ G1 ) (Fig. 1a ), sandwiched between the porphyrins with a high association constant ( K a = ca. 2.2 × 10 9 M −1 in CH 3 CN). Thus, a series of naphthalenemonoimide ( NMI )-based enantiopure and/or racemic guests G2 – G8 (Fig. 1a ) were synthesized by the reaction of G1 with various kinds of chiral primary amines (see Supplementary Methods). Water-mediated racemization of the helicate The water-mediated racemization kinetics of ( M )- 1 TBA2 was first investigated by circular dichroism (CD) spectroscopy in aprotic polar solvents such as dimethyl sulfoxide (DMSO) (Supplementary Fig. 1 ). As anticipated, the intense positive-bisignate CD signal of ( M )- 1 TBA2 [36] remained unchanged after heating at 70 °C for 24 h in anhydrous DMSO, whereas its CD intensity gradually decreased with time at high temperatures (70–110 °C) as a result of the racemization in the presence of water (ca. 500 equivalents to ( M )- 1 TBA2 ) (Supplementary Fig. 1a,b ). The pseudo-first-order rate constants ( k rac , s −1 ) and half-life time periods ( t 1/2 , h) for the racemization of ( M )- 1 TBA2 estimated by the CD intensity changes at different temperatures provided the thermodynamic parameters based on the Arrhenius and Eyring plots of the kinetic data (Supplementary Fig. 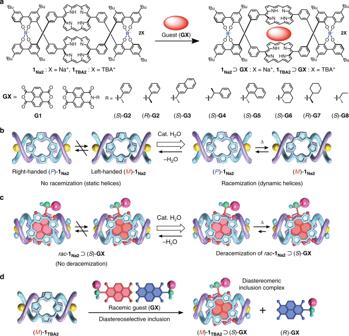Fig. 1 Deracemization and diastereoselective inclusion complexation of double-stranded spiroborate helicates.aChemical structures of double-stranded bisporphyrin helicates1X2(X = Na+or TBA+) and their inclusion complexation with achiral (G1) or chiral (G2–G8) electron-deficient aromatic guests.b,cSchematic representations of water-catalyzed racemization ofrac-1Na2(b), deracemization ofrac-1Na2upon the inclusion complex formation with an enantiopure guest (c), and diastereoselective inclusion complexation of racemic guest with left-handed (M)-1TBA2(d) 1c–e ), which are summarized in Supplementary Table 1 . Interestingly, the inclusion complex formation of ( M )- 1 TBA2 with G1 resulted in an increase in the racemization rates of ( M )- 1 TBA2 ⊃ G1 as compared to those of the free ( M )- 1 TBA2 under the same conditions (Supplementary Fig. 2 ), probably due to the B–O bond strain at the spiroborate moieties of the helicate [47] that increases upon complexation with G1 . Such steric strain within the spiroborate helicate could be relaxed during the water-catalyzed B–O bond cleavage reactions at the spiroborate groups, leading to a significant increase in the activation entropy (Δ S ‡ ) for the racemization from −42 ± 11 (( M )- 1 TBA2 ) to 4 ± 20 J mol −1 (( M )- 1 TBA2 ⊃ G1 ) (Supplementary Table 1 ). Intermolecular hydrogen bond formation between the included G1 and water, which may accelerate the water-catalyzed racemization of the ( M )- 1 TBA2 ⊃ G1 inclusion complex, could also be taken into consideration. We note that inversion of the helicity of the helicate 1 requires simultaneous cleavages of one of the four B–O bonds at each spiroborate group by the formation of an achiral meso intermediate, followed by reforming of the spiroborated ( P )- or ( M )-helicate (Supplementary Fig. 1f ). Helix-sense-selective deracemization of racemic helicate The deracemization of rac - 1 Na2 was then performed in the presence of various chiral guests (3 equivalents) (( R )- or ( S )- G2 – G8 , Fig. 1a ) in various solvents containing a small amount of water at 80 °C for an appropriate length of time until reaching an equilibrium state. We chose this temperature (80 °C) based on the relationship between the diastereomeric excess (d.e.) of the optically-active 1 Na2 ( derac - 1 Na2 ) complexed with ( S )- G2 in DMSO- d 6 and the time required to reach an equilibrium state at various temperatures (Supplementary Fig. 3 ), although higher d.e. values will be obtained by a prolonged heating at lower temperatures. The d.e. values of derac - 1 Na2 complexed with chiral guests (( P )- and ( M )- 1 Na2 ⊃ chiral guest) were determined based on their 1 H nuclear magnetic resonance (NMR) spectra except for those with G6 and G7 (Table 1 , runs 1–8 and Fig. 2a and Supplementary Fig. 4 ). The chiral guests included in the derac - 1 Na2 were then replaced by the achiral G1 to produce the corresponding enantiomeric derac - 1 Na2 ⊃ G1 complexes (for detailed experimental procedures, see Methods) and their enantiomeric excess (e.e.) values that correspond to their helical sense excesses of the derac - 1 Na2 and its helical handedness ( P or M ) were determined by their CD spectra (Fig. 2b ) based on the molar ellipticity at 419 nm (Δ ε 419 ) and its sign of the one-handed helical ( M )- 1 TBA2 ⊃ G1 complex (e.e. >99%) [47] as the base value, respectively (Table 1 , runs 1–8). The complete replacement of the guests with G1 was confirmed by model experiments (Supplementary Fig. 5 ). The CD spectra of the derac - 1 Na2 ⊃ G1 complexes assisted by ( R )- and ( S )- G2 displayed perfect mirror images with almost similar e.e. values of 44% and 47%, respectively, which are in good agreement with the corresponding d.e. values (44%) estimated by 1 H NMR (Table 1 , runs 1 and 2). Table 1 Deracemization of rac -1 Na2 with chiral guests in various solvents at 80 °C Full size table Fig. 2 Deracemization of rac - 1 Na2 upon inclusion complexation with various enantiopure guests in various solvents. a Partial 1 H NMR spectra of mixtures of rac - 1 Na2 (0.50 mM) with ( S )- G2 , ( S )- G3 , ( S )- G4 , and ( S )- G5 ([guest]/[ 1 Na2 ] = 3) in DMSO- d 6 measured at ambient temperature after heating at 80 °C for 24–48 h. [H 2 O]/[ 1 Na2 ] = ca. 5–150. For the assignment of ( P )- and ( M )-helicity, see the text. b CD and absorption spectra of derac - 1 Na2 (0.20 mM) in the presence of 3 equivalents of achiral G1 measured in CH 3 CN/DMSO- d 6 (ca. 29/1, v/v) or CH 3 CN/DIPF (ca. 29/1, v/v) at 25 °C after deracemization of rac - 1 Na2 upon inclusion complexation with GX ([guest]/[ 1 Na2 ] = 3) in DMSO- d 6 (for G2 – G8 ) or DIPF (for ( S )- G3 ) at 80 °C for 24–48 h. For detailed experimental procedures, see Methods (Procedure A). c Partial 1 H NMR spectra of 1 Na2 (0.50 mM) with ( S )- G3 ([( S )- G3 ]/[ 1 Na2 ] = 3) in CD 3 CN, acetone- d 6 , and THF- d 8 measured at ambient temperature after heating at 80 °C for 26–266 h. [H 2 O]/[( M )- 1 TBA2 ] = ca. 5–20. Asterisk denotes the protons from unknown impurities Full size image The deracemization results of rac - 1 Na2 assisted by the chiral guests ( G2 – G8 ) in DMSO- d 6 at 80 °C revealed that the helix-sense ( P or M ) and its helix-sense excess (% e.e.) of the produced derac - 1 Na2 were significantly affected by the structures of the chiral pendant groups of the NMI -based guests (Table 1 , runs 1–8). The chiral guests bearing bulky aromatic pendants, such as the 1-phenylethtyl (( S )- and ( R )- G2 ) and 1-(2-naphthyl)ethyl (( S )- G3 ) groups, afforded an optically-active derac - 1 Na2 with an appreciable level of helix-sense selectivity at 80 °C (47% and 55% e.e., respectively), while those carrying aromatic, but flexible (( S )- G4 ) and aliphatic (( R )- G7 and ( S )- G8 ) pendants produced the derac - 1 Na2 with low % e.e. (10%, 28%, and 2%, respectively). Surprisingly, the chiral aromatic guests ( S )- G5 and ( S )- G6 that are similar to G3 and G2 in their structures afforded a slightly enantio-enriched derac - 1 Na2 with 28% and 6% e.e., respectively. Among the chiral guests, ( S )- G2 –( S )- G5 produced the same ( M )-rich derac - 1 Na2 , while ( S )- G6 , ( R )- G7 , and ( S )- G8 afforded derac - 1 Na2 with the opposite handedness. These results suggest that the NMI -based guests with moderately steric chiral aromatic pendant groups capable of interacting with the rac - 1 Na2 in a diastereoselective fashion are required for achieving a highly helix-sense-selective deracemization of the rac - 1 Na2 (see the next section). We next investigated the solvent effect on the deracemization of rac - 1 Na2 assisted by ( S )- G2 and ( S )- G3 using various solvents at 80 °C under identical conditions in DMSO- d 6 (Table 1 ). The helix-sense excesses of the produced derac - 1 Na2 were estimated in the same way by CD and 1 H NMR (Fig. 2b, c and Supplementary Figs. 6 and 7 ). Both of the guests preferentially afforded the ( M )-rich derac - 1 Na2 independent of the solvents (Table 1 , runs 9, 10, 12, 13, 15–26), whereas the helix-sense-selectivities were highly dependent on the solvents, producing relatively high ( M )-enriched derac - 1 Na2 in THF, DMF, DEF, and DIPF (e.e. >50%) with up to 72% e.e. in DIPF when ( S )- G3 was used as the guest (Table 1 , run 26). Interestingly, the e.e. values of the derac - 1 Na2 produced in similar solvents (DMF, DEF, and DIPF) increased with an increase in the N , N -disubstituted alkyl chain length (Table 1 , runs 21–26). A similar increase in the e.e. value was also observed when IBN (43–44% e.e.) was used instead of CD 3 CN (12–16% e.e.) as the solvent (Table 1 , runs 9, 10, 17, and 18), indicating an important role of the solvent structures as well as its polarity. The inclusion complex of rac - 1 Na2 ⊃ ( S )- G3 could be completely separated into rac - 1 Na2 and ( S )- G3 by size-exclusion chromatography (SEC) using DMF as the eluent (Supplementary Fig. 8 ), which enables us to recover the optically-active 1 Na2 for further applications, and at the same time, chiral guests for recycle. Encouraged by this straightforward separation, a scaled-up deracemization reaction of rac - 1 Na2 (7.9 mg, 3.6 μmol) with ( S )- G3 (3 equivalents) was performed in DIPF at 80 °C for 24 h, producing an optically-active derac - 1 Na2 ⊃ ( S )- G3 with 74% d.e. (Supplementary Fig. 9 ). Subsequent SEC isolation afforded derac - 1 Na2 and ( S )- G3 in excellent yields of 91% and 93% with >70% and 99% e.e., respectively. Diastereoselective encapsulation of racemic guests We anticipated that the observed helix-sense-selective deracemization of the rac - 1 Na2 with chiral guests was mostly due to differential inclusion complexation of an enantiopure guest (( S )- G2 for example) toward rac - 1 Na2 with an appreciable level of diastereoselectivity. To confirm this and also to disclose an energetic driving force for the helix-sense-selectivity during the deracemization process, we investigated the chiral recognition ability [13] , [46] , [50] , [51] , [52] , [53] , [54] , [55] of the one-handed helical ( M )- 1 TBA2 toward racemic guests ( G2 – G4 ) in various solvents at different temperatures during the inclusion complexation in the bisporphyrin cavity of ( M )- 1 TBA2 by 1 H NMR spectroscopy (Fig. 1d ). Upon mixing ( M )- 1 TBA2 and ( R )- or ( S )- G2 in a 1:1 molar ratio in THF- d 8 at 25 °C, the 1:1 inclusion complex was quantitatively produced. The 1 H NMR signals of the ( M )- 1 TBA2 were split into two sets of new signals as a result of desymmetrization of the pseudo- D 2 -symmetric structure of 1 TBA2 upon the inclusion complexation with the non-symmetric NMI -based guests (Fig. 3a ). Thus, a mixture of ( M )- 1 TBA2 with 3 equivalents of rac - G2 in THF- d 8 showed the signals corresponding to the diastereomers ( M )- 1 TBA2 ⊃ ( R )- G2 and ( M )- 1 TBA2 ⊃ ( S )- G2 with 66% d.e. ( S rich) (Fig. 3b ), which is very consistent with the diastereoselectivity (73% d.e.) calculated by using the association constants of ( M )- 1 TBA2 with ( S )- G2 (ca. 2.4 × 10 6 M −1 ) and ( R )- G2 (ca. 3.7 × 10 5 M −1 ) estimated by the fluorescence titration experiments (Supplementary Fig. 10 ). The diastereoselectivity of ( M )- 1 TBA2 with rac - G2 was highly dependent on the solvents (Fig. 3b and Supplementary Fig. 12 ) being relevant to the deracemization results (Table 1 ), and the % d.e. value ( S rich) at 25 °C drastically decreased in the following order: THF- d 8 (66) > DMF- d 7 (48) > acetone- d 6 (45) > DMSO- d 6 (39) > CD 3 CN (8), accompanied by chirality inversion of the G2 preferentially included in ( M )- 1 TBA2 in CD 3 CN (Fig. 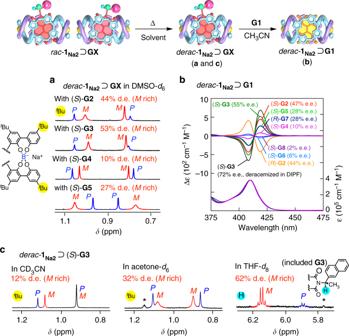Fig. 2 Deracemization ofrac-1Na2upon inclusion complexation with various enantiopure guests in various solvents.aPartial1H NMR spectra of mixtures ofrac-1Na2(0.50 mM) with (S)-G2, (S)-G3, (S)-G4, and (S)-G5([guest]/[1Na2] = 3) in DMSO-d6measured at ambient temperature after heating at 80 °C for 24–48 h. [H2O]/[1Na2] = ca. 5–150. For the assignment of (P)- and (M)-helicity, see the text.bCD and absorption spectra ofderac-1Na2(0.20 mM) in the presence of 3 equivalents of achiralG1measured in CH3CN/DMSO-d6(ca. 29/1, v/v) or CH3CN/DIPF (ca. 29/1, v/v) at 25 °C after deracemization ofrac-1Na2upon inclusion complexation withGX([guest]/[1Na2] = 3) in DMSO-d6(forG2–G8) or DIPF (for (S)-G3) at 80 °C for 24–48 h. For detailed experimental procedures, see Methods (Procedure A).cPartial1H NMR spectra of1Na2(0.50 mM) with (S)-G3([(S)-G3]/[1Na2] = 3) in CD3CN, acetone-d6, and THF-d8measured at ambient temperature after heating at 80 °C for 26–266 h. [H2O]/[(M)-1TBA2] = ca. 5–20. Asterisk denotes the protons from unknown impurities 3b and Supplementary Table 2 ), which is also consistent with the diastereoselectivity (4% d.e.) calculated by the association constants of ( M )- 1 TBA2 with ( S )- G2 (ca. 5.9 × 10 6 M −1 ) and ( R )- G2 (ca. 6.4 × 10 6 M −1 ) (Supplementary Fig. 11 ). Such a solvent-induced switching of the diastereoselectivity during the inclusion complexation of the racemic guests with ( M )- 1 TBA2 was also observed by changing the temperature (see below). Fig. 3 Diastereoselective inclusion complexation between ( M )- 1 TBA2 and rac - G2 or rac - G3 . a Schematic representations of diastereoselective inclusion complexation of racemic guest with left-handed ( M )- 1 TBA2 . Partial 1 H NMR spectra (500 MHz, 0.40 mM, 25 °C) of ( M )- 1 TBA2 in the absence (i) and presence of 1 equivalent of ( S )- G2 (ii), and ( R )- G2 (iii) in THF- d 8 . b Partial 1 H NMR spectra (500 MHz, 0.40 mM, 25 °C) of ( M )- 1 TBA2 in the presence of 3 equivalents of rac - G2 in CD 3 CN, THF- d 8 , acetone- d 6 , DMF- d 7 , and DMSO- d 6 . The diastereomeric excess (d.e.) values were estimated by the integral ratio of the t Bu or methine proton signals derived from the diastereomeric inclusion complexes ( M )- 1 TBA2 ⊃ ( S )- G2 (red closed circle) and ( M )- 1 TBA2 ⊃ ( R )- G2 (blue closed circle). Hash and asterisk denote the protons from TBA and unknown impurities, respectively. The signals of ( M )- 1 TBA2 , ( M )- 1 TBA2 ⊃ ( R )- G2 , and ( M )- 1 TBA2 ⊃ ( S )- G2 in THF- d 8 were assigned by two-dimensional gradient correlation spectroscopy (gCOSY) and rotating frame nuclear Overhauser enhancement spectroscopy (ROESY) measurements (Supplementary Figs. 20 – 35 ). c Variable temperature (VT) partial 1 H NMR spectra (500 MHz, 0.40 mM) of ( M )- 1 TBA2 in the presence of 3 equivalents of rac - G3 in THF- d 8 from −55 to 55 °C Full size image The diastereoselectivities of ( M )- 1 TBA2 with rac - G2 in THF- d 8 and CD 3 CN were significantly dependent on the temperature (Supplementary Table 2 ), and the d.e. value gradually increased with the decreasing temperature and reached 94 ( S -rich) and 42% ( R -rich) at −75 and −35 °C, respectively, while the chirality of the enriched enantiomer of G2 in the ( M )- 1 TBA2 was inverted in CD 3 CN at temperatures below 40 °C (Supplementary Fig. 13 ). A similar temperature-dependent enhancement of the diastereoselectivity of ( M )- 1 TBA2 in THF- d 8 and CD 3 CN together with inversion of the diastereoselectivity in CD 3 CN was also observed for rac - G3 (Supplementary Fig. 14 ). Of particular interest is that ( M )- 1 TBA2 completely recognized the chirality of G3 enantiomers to form the inclusion complex only with ( S )- G3 (>99% d.e.) in THF- d 8 at below −50 °C (Fig. 3c and Supplementary Table 2 ). In contrast, ( M )- 1 TBA2 was almost temperature-independent with moderate ( R )- and ( S )-selectivities to rac - G4 carrying an aromatic, but a flexible 2-phenylpropyl pendant group in CD 3 CN and THF- d 8 , respectively (Supplementary Fig. 15 and Supplementary Table 2 ). Thus, the solvent and chiral guest-dependent changes in the diastereoselectivity of ( M )- 1 TBA2 toward racemic chiral guests at high temperatures seem to be relevant to the deracemization results of rac - 1 Na2 upon complexation with the enantiopure guests (Table 1 , runs 9–14 and Supplementary Table 2 ). The observed differences in the diastereoselectivities of ( M )- 1 TBA2 toward racemic guests G2 – G4 indicated the important role of the position of the aromatic pendant groups in its diastereoselective inclusion complexation. We then constructed the inclusion model structures for a pair of the diastereomers, ( M )- 1 complexed with ( R )- and ( S )- G2 (Fig. 4a, b and Supplementary Figs. 17 and 18 ) as well as those with ( R )- and ( S )- G4 (Supplementary Fig. 19 ) based on the analogous crystal structure of the inclusion complex of rac - 1 Na2 ⊃ G1 , in which the achiral symmetric G1 is sandwiched between the bisporphyrin in a parallel fashion via face-to-face stacking interactions [36] , followed by the density functional theory (DFT) calculations (Supplementary Methods). The sandwich structures of ( M )- 1 TBA2 ⊃ G2 and ( M )- 1 TBA2 ⊃ G4 were supported by the 1 H two-dimensional (2D) NMR experiments (Supplementary Figs. 30 – 47 ). The locations of ( R )- and ( S )- G2 complexed with ( M )- 1 are best illustrated in Fig. 4a, b , in which the NMI cores are intercalated between the porphyrins with different orientations of the NMI cores. As a result, the pendant phenyl group of ( S )- G2 is oriented almost perpendicular to the porphyrin rings (edge-to-face arrangement) so as to position above the meso -proton ( meso -H (H a’A )) and its neighboring β -proton ( β -H: H b2’A ) of the porphyrin in Fig. 4a , although that of ( R )- G2 is positioned close to and above the β -protons ( β -H: H b1’A and H c1’A ) instead of the H a’A and H b2’A protons (Fig. 4b ). These spatial arrangements of the pendant phenyl groups suggest possible edge-to-face CH–π interactions [56] , [57] between the pendant phenyl groups of ( S )- and ( R )- G2 and the meso -H and/or β -H protons that can function more effectively for the ( M )- 1 ⊃ ( S )- G2 complex, leading to the observed ( S )-selective inclusion complexation with ( M )- 1 in various solvents except for CD 3 CN at or below 40 °C (Fig. 3b and Supplementary Table 2 ). These energy-minimized models explain the significant upfield shifts of the specific meso -H and β -H protons of the porphyrin rings of ( M )- 1 TBA2 complexed with ( S )- and ( R )- G2 (Fig. 4c(i, ii) and Supplementary Figs. 24 and 25 ; see below) and are supported by the intermolecular nuclear Overhauser effect (NOE) cross-peaks observed between the meso -H and β -H protons of the porphyrin rings of ( M )- 1 TBA2 and the aromatic protons of ( S )- G2 at low temperature (Fig. 4d and Supplementary Fig. 26 ). Fig. 4 Mechanism of diastereoselective inclusion complexation of racemic guests with ( M )- 1 TBA2 . Top and side views of the energy-minimized inclusion complex structures of ( M )- 1 2 − ⊃ ( S )- G2 ( a ) and ( M )- 1 2 − ⊃ ( R )- G2 ( b ) with different geometries ( A opt and B opt ) (see Supplementary Figs. 16 and 17 ), obtained by the DFT calculations with the D3 dispersion correction (for more details, see Supplementary Methods). 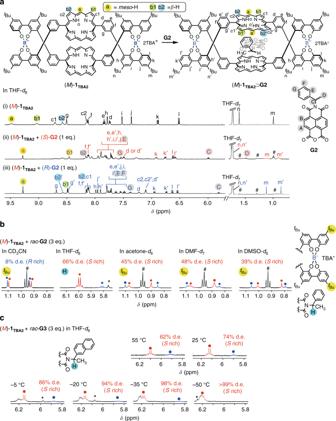Fig. 3 Diastereoselective inclusion complexation between (M)-1TBA2andrac-G2orrac-G3.aSchematic representations of diastereoselective inclusion complexation of racemic guest with left-handed (M)-1TBA2. Partial1H NMR spectra (500 MHz, 0.40 mM, 25 °C) of (M)-1TBA2in the absence (i) and presence of 1 equivalent of (S)-G2(ii), and (R)-G2(iii) in THF-d8.bPartial1H NMR spectra (500 MHz, 0.40 mM, 25 °C) of (M)-1TBA2in the presence of 3 equivalents ofrac-G2in CD3CN, THF-d8, acetone-d6, DMF-d7, and DMSO-d6. The diastereomeric excess (d.e.) values were estimated by the integral ratio of thetBu or methine proton signals derived from the diastereomeric inclusion complexes (M)-1TBA2⊃(S)-G2(red closed circle) and (M)-1TBA2⊃(R)-G2(blue closed circle). Hash and asterisk denote the protons from TBA and unknown impurities, respectively. The signals of (M)-1TBA2, (M)-1TBA2⊃(R)-G2, and (M)-1TBA2⊃(S)-G2in THF-d8were assigned by two-dimensional gradient correlation spectroscopy (gCOSY) and rotating frame nuclear Overhauser enhancement spectroscopy (ROESY) measurements (Supplementary Figs.20–35).cVariable temperature (VT) partial1H NMR spectra (500 MHz, 0.40 mM) of (M)-1TBA2in the presence of 3 equivalents ofrac-G3in THF-d8from −55 to 55 °C The energy difference (Δ E stb ) values are also shown (see also Supplementary Table 3 ). Hydrogen atoms except for meso - and β -protons of the porphyrin rings and G2 are omitted for clarity. The t Bu groups were replaced with hydrogen to simplify the calculations. The included guests are highlighted as a space-filling model. Hydrogen atoms except for meso - and β -protons of the porphyrin rings and G2 are omitted for clarity. c Partial 1 H NMR spectra (500 MHz, 0.40 mM, −50 °C) of ( M )- 1 TBA2 in the presence of 1 equivalent of ( S )- G2 (i), ( R )- G2 (ii), ( S )- G4 (iii), and ( R )- G4 (iv) in THF- d 8 . d Partial NOESY spectra (500 MHz, 0.40 mM, mixing time = 800 ms) of ( M )- 1 2 − ⊃ ( S )- G2 in THF- d 8 at −50 °C Full size image In contrast, the phenyl groups of ( R )- and ( S )- G4 are located far from the meso -H and β -H protons, so that effective CH–π interactions may not be anticipated (Supplementary Fig. 19 ) as supported by slight upfield shifts of the meso -H and β -H protons compared to those of ( M )- 1 TBA2 complexed with G2 due to lack of the ring current effect of the pendant phenyl groups of G4 , thus showing moderate diastereoselectivities (18–38% d.e.) with opposite ( R )- and ( S )- G4 selectivities in CD 3 CN and THF- d 8 , respectively (Supplementary Table 2 ). These results are in good agreement with those of the deracemization of rac - 1 Na2 complexed with ( S )- G4 in CD 3 CN and THF- d 8 , giving derac - 1 Na2 with opposite P and M helicities, respectively (Table 1 , runs 11 and 14). This speculation was supported by the remarkable differences in the temperature-dependent 1 H NMR spectral changes of ( M )- 1 TBA2 complexed between G2 and G4 in THF- d 8 (Supplementary Figs. 20 – 22 ). Upon complexation with the non-symmetric chiral G2 and G4 , all of the aromatic and porphyrin proton signals of ( M )- 1 TBA2 including the meso -H (a) and β -H (b 1 and b 2 ) signals of the porphyrin rings split into two sets of non-equivalent signals independent of the guests and solvents (CD 3 CN and THF- d 8 ) at 25 °C (Fig. 3a and Supplementary Figs. 23 and 28 ) except for the ( M )- 1 TBA2 ⊃ G2 complex in THF- d 8 ; the specific meso -H (a’) and β -H (b 1’ and b 2’ ) signals of the porphyrin rings were not observed at 25 °C due to broadening of the signals (Fig. 3a ). In addition, the aromatic and porphyrin proton signals of the ( M )- 1 TBA2 ⊃ ( S )- G2 complex in THF- d 8 were significantly broadened when compared to those of its diastereomer ( M )- 1 TBA2 ⊃ ( R )- G2 (Fig. 3a ) due to the relatively slow rotation of the ( S )-1-phenylethyl group around the N–C α bond of the included ( S )- G2 at 25 °C (see below). Upon cooling to a low temperature, the N–C α bond rotation of the ( M )- 1 TBA2 ⊃ ( S )- G2 complex appeared to be further restricted from free rotation and finally frozen because more effective edge-to-face CH–π contacts act as a molecular brake [58] that prevents rotation around the N–C α bond of ( S )- G2 sandwiched between the two porphyrins, thereby leading to further splitting of the porphyrin and aromatic protons as well as the tert -butyl ( t Bu) protons of the helicate in THF- d 8 below −5 °C (Supplementary Fig. 21a ; for proton peak splitting diagrams for the meso -H and β -H protons of ( M )- 1 TBA2 upon complexation with non-symmetric chiral guests, see Supplementary Fig. 20 ). Similar splitting of the proton resonances was also observed for the ( M )- 1 TBA2 ⊃ ( R )- G2 complex, but appeared below −50 °C (Supplementary Fig. 21b ). The chemical shift difference between the two newly-appeared meso -H signals (H a’A and H a’B ) (Δδ meso ) of the porphyrin rings of ( M )- 1 TBA2 complexed with ( S )- G2 (1.64 ppm at −25 °C) in THF- d 8 was significantly greater than that with ( R )- G2 (0.66 ppm at −50 °C), whereas the corresponding chemical shift difference between the β -H signals (H b1’A and H b1’B ) (Δδ β ) was ca. 0.04 ppm for ( S )- G2 at −25 °C that was smaller than 1.21 ppm for ( R )- G2 at −50 °C (Supplementary Figs. 24 and 25 ). These results are consistent with the calculated structural models (Fig. 4a, b ) with respect to the relative orientations of the pendant phenyl groups of ( R )- and ( S )- G2 complexed with ( M )- 1 2− . The 2D EXSY (exchange spectroscopy) spectra of the ( M )- 1 TBA2 ⊃ ( S )- G2 complex acquired at different mixing times in THF- d 8 at −25 °C showed a series of chemical exchange cross-peaks between the two porphyrin protons due to slow rotation of the ( S )-1-phenylethyl group (Supplementary Fig. 29 ), and the apparent exchange rate constant (rotation rate) was estimated to be 5.97 s −1 (Supplementary Methods and Supplementary Fig. 29 ). In contrast, the ( M )- 1 TBA2 ⊃ ( R )- G2 complex exhibited no chemical exchange cross-peaks in THF- d 8 at −25 °C due to fast rotation of the ( R )-1-phenylethyl group, but showing the cross-peaks at −50 °C (Supplementary Fig. 25 ). In sharp contrast, ( R )- and ( S )- G4 bearing a methylene-linked flexible pendant did not show such non-equivalent splitting of the proton signals when complexed with ( M )- 1 TBA2 in THF- d 8 even at low temperatures because of almost the free rotation of the flexible pendant group (Supplementary Fig. 22 ), which clearly revealed the more favorable edge-to-face CH–π contacts of ( M )- 1 TBA2 with G2 than those with G4 in THF- d 8 , thereby showing a much higher diastereoselectivity of ( M )- 1 TBA2 toward rac - G2 than rac - G4 in THF- d 8 (Supplementary Table 2 ). In addition, the N–C α bond rotation of the ( M )- 1 TBA2 ⊃ ( S )- G2 complex became much faster in CD 3 CN comparable to that of the ( M )- 1 TBA2 ⊃ ( R )- and ( S )- G4 complexes in THF- d 8 judging from their variable-temperature 1 H NMR spectral changes (Supplementary Figs. 22 and 27 ). 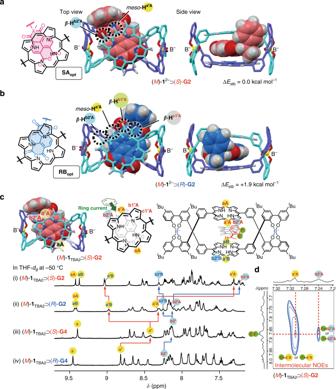Fig. 4 Mechanism of diastereoselective inclusion complexation of racemic guests with (M)-1TBA2. Top and side views of the energy-minimized inclusion complex structures of (M)-12−⊃(S)-G2(a) and (M)-12−⊃(R)-G2(b) with different geometries (AoptandBopt) (see Supplementary Figs.16and17), obtained by the DFT calculations with the D3 dispersion correction (for more details, see Supplementary Methods). The energy difference (ΔEstb) values are also shown (see also Supplementary Table3). Hydrogen atoms except formeso- andβ-protons of the porphyrin rings andG2are omitted for clarity. ThetBu groups were replaced with hydrogen to simplify the calculations. The included guests are highlighted as a space-filling model. Hydrogen atoms except formeso- andβ-protons of the porphyrin rings andG2are omitted for clarity.cPartial1H NMR spectra (500 MHz, 0.40 mM, −50 °C) of (M)-1TBA2in the presence of 1 equivalent of (S)-G2(i), (R)-G2(ii), (S)-G4(iii), and (R)-G4(iv) in THF-d8.dPartial NOESY spectra (500 MHz, 0.40 mM, mixing time = 800 ms) of (M)-12−⊃(S)-G2in THF-d8at −50 °C Therefore, the diastereoselectivity of ( M )- 1 TBA2 toward rac - G2 in CD 3 CN significantly decreased, suggesting the important role of the CH–π interactions in the diastereoselective inclusion complexation [59] that are highly dependent on the solvents. These 1 H NMR analyses combined with the DFT calculated structures of the complexes revealed that the remarkable solvent- and guest-dependent changes in the diastereoselective inclusion complexation of the racemic guests in the ( M )- 1 TBA2 cavity appear to mainly rely on the edge-to-face CH-π interactions between the pendant phenyl rings of the guests and the protons at the meso and its neighboring β -positions of the porphyrin rings, because the CH–π interactions are sensitive to the solvents [60] , [61] and significantly contribute to the molecular and chiral recognition events [56] , [57] , [59] . 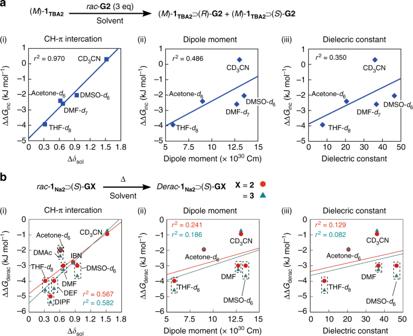Fig. 5 Mechanism of deracemization ofrac-1Na2with chiral guests.aPlots of ΔΔGinc(the difference in free energy for the diastereomeric inclusion complexation between (M)-1TBA2and (S)-G2/(R)-G2at 25 °C) against Δδsol(Supplementary Table5) (i), dipole moment (ii), and dielectric constant (iii) of the solvents.bPlots of ΔΔGderac(the difference in free energy for the diastereoselective deracemization ofrac-1Na2with (S)-G2and (S)-G3at 80 °C) against Δδsol(i), dipole moment (ii), and dielectric constant (iii) of the solvents. Source data of (a) and (b) are provided as aSource Datafile According to the literature [60] , the difference in the proton chemical shifts (Δ δ sol ) of given solvents between in deuterated aromatic and non-aromatic solvents, such as C 6 D 6 and CDCl 3 , respectively, can be used as a measure to evaluate the CH–π interaction capabilities of the solvent molecules (Supplementary Table 5 ); the solvents with a higher Δ δ sol value, such as CH 3 CN, tend to strongly interact with aromatic molecules, and hence, the CH–π interactions between the host–guest complexes will be hindered. The difference in free energy (ΔΔ G inc ) upon diastereomeric inclusion complexation between ( M )- 1 TBA2 and ( S )-/( R )- G2 in various solvents at 25 °C was then calculated using the d.e. value in each solvent (Supplementary Table 2 ) then plotted versus the Δ δ sol values, which gave an almost straight line (Fig. 5a ) (i), suggesting the very important role of the CH–π interactions in the diastereoselective inclusion complexation. For comparison, the ΔΔ G inc values were also plotted versus other solvent parameters, such as the dipole moment (ii) and dielectric constant (iii), which did not show a good correlation (Fig. 5a ). Fig. 5 Mechanism of deracemization of rac - 1 Na2 with chiral guests. a Plots of ΔΔ G inc (the difference in free energy for the diastereomeric inclusion complexation between ( M )- 1 TBA2 and ( S )- G2 /( R )- G2 at 25 °C) against Δ δ sol (Supplementary Table 5 ) (i), dipole moment (ii), and dielectric constant (iii) of the solvents. b Plots of ΔΔ G derac (the difference in free energy for the diastereoselective deracemization of rac - 1 Na2 with ( S )- G2 and ( S )- G3 at 80 °C) against Δ δ sol (i), dipole moment (ii), and dielectric constant (iii) of the solvents. Source data of ( a ) and ( b ) are provided as a Source Data file Full size image In the same way, the calculated difference in free energy (ΔΔ G derac ) in the helix-sense selective deracemization of rac - 1 Na2 assisted by ( S )- G2 and ( S )- G3 in various solvents at 80 °C based on the d.e. values in Table 1 was plotted versus the Δ δ sol values (i), dipole moment (ii), and dielectric constant (iii). Among them, the plot versus the Δ δ sol values gave an approximate correlation between them (Fig. 5b ), indicating the key role of the CH–π interactions being relevant to the diastereoselective inclusion complexation of enantiopure guests toward rac - 1 Na . These results imply that if the deracemization experiment is carried out at lower temperatures in specific solvents, such as THF, the helix-sense selectivity may be significantly improved, although it will take a longer time to reach an equilibrium, while it may be possible when an acid instead of water is used as a catalyst for the catalytic B–O bond cleavage/reformation of the spiroborate groups of the helicate. We have found that a racemic double-stranded spiroborate helicate deracemizes via water-mediated B–O bond cleavage/reformation of the spiroborate groups that proceeds in a highly helix-sense selective manner upon diastereoselective inclusion complexation of an enantiopure aromatic guest between the porphyrin rings linked to the racemic helicate. The double-stranded helicate is kinetically inert toward racemization in the absence of water, but its interconversion between the enantiomeric double helices can be switched on and off by the addition and removal of water. Attractive CH–π interactions between the pendant aromatic group of the encapsulated chiral guests and the porphyrin protons of the helicate are indispensable for an efficient diastereoselective inclusion complexation, thus leading to an excellent helix-sense selectivity during the water-mediated deracemization. The present findings imply that analogous dynamically racemic helicates and supramolecules can be converted into the corresponding kinetically-stable enantiomers via deracemization in the presence of chiral guests through noncovalent chiral interactions. General procedures for the deracemization Procedure A : For the deracemization of rac - 1 Na2 upon inclusion complexation with ( S )- G2 in DIPF, stock solutions of rac -1 Na2 (0.50 mM) (solution I) and ( S )- G2 (solution II) (2.0 mM) were prepared in CH 3 CN. Aliquots of I (0.35 µmol, 700 µL) and II (1.05 µmol, 525 µL) were added to a vial, then the solvent was removed under reduced pressure. The vial containing rac -1 Na2 and 3 equivalents of ( S )- G2 was sealed with a rubber septum, and to this was added distilled DIPF (700 µL) using a syringe under nitrogen. The DIPF solution was then heated to 80 °C for the appropriate length of time (24 h) until reaching an equilibrium state. The H 2 O content in the reaction mixture was estimated by measuring the 1 H NMR spectrum of the mixture after dilution with dried DMSO- d 6 (DIPF/DMSO- d 6 = 1/70, v/v). The reaction progress was monitored at an appropriate time interval by CD and absorption measurements of the reaction mixture after cooling to room temperature, then diluted 30-fold with a CH 3 CN solution containing 3 equivalents of the achiral G1 . The percent e.e. value of the deracemized 1 Na2 complexed with G1 was then estimated based on the following equation: 
    e.e. ( %) = Δε_419/Δε_419( max)× 100
 where Δε 419 and Δε 419(max) are the CD intensities (1st Cotton effect at 419 nm) of the derac - 1 Na2 ⊃ G1 and enantiopure ( M )- 1 TBA2 ⊃ G1 (e.e. >99%), respectively. In the same way, the deracemization of rac -1 Na2 upon inclusion complexation with enantiopure guests in various solvents were performed and the results are summarized in Table 1 . Procedure B : The deracemization progress was also directly monitored by 1 H NMR spectroscopy in CD 3 CN, THF- d 8 , DMSO- d 6 , and acetone- d 6 . For the deracemization of rac -1 Na2 upon inclusion complexation with G2 in DMSO- d 6 , stock solutions of rac -1 Na2 (0.50 mM) (solution I) and ( S )- G2 (solution II) (2.0 mM) were prepared in CH 3 CN. Aliquots of I (0.35 µmol, 700 µL) and II (1.05 µmol, 525 µL) were added to an NMR tube, then the solvent was removed under reduced pressure. The NMR tube was sealed with a rubber septum, then subjected to three evacuation/nitrogen fill cycles. To this was added 700 µL of DMSO- d 6 via a syringe. The tube was then sealed with a small flame and the solution was heated to 80 °C for an appropriate length of time (38 h) until reaching an equilibrium state. The reaction progress was monitored at an appropriate time interval by 1 H NMR measurements of the reaction mixture after cooling to 25 °C. The d.e. value of the deracemized 1 Na2 was estimated by the integral ratio of the diastereomeric t Bu signals derived from ( M )- 1 Na2 ⊃ ( S )- G2 and ( P )- 1 Na2 ⊃ ( S )- G2 (Fig. 2a ). In the same way, the deracemization of rac -1 Na2 upon inclusion complexation with enantiopure guests in various solvents, such as CD 3 CN, acetone- d 6 , and THF- d 8 , was performed at 80 °C and the results are summarized in Table 1 .